Achieving a long-lived high-beta plasma state by energetic beam injection Developing a stable plasma state with high-beta (ratio of plasma to magnetic pressures) is of critical importance for an economic magnetic fusion reactor. At the forefront of this endeavour is the field-reversed configuration. Here we demonstrate the kinetic stabilizing effect of fast ions on a disruptive magneto-hydrodynamic instability, known as a tilt mode, which poses a central obstacle to further field-reversed configuration development, by energetic beam injection. This technique, combined with the synergistic effect of active plasma boundary control, enables a fully stable ultra-high-beta (approaching 100%) plasma with a long lifetime. Nuclear fusion potentially offers a clean, environment-friendly and intrinsically safe energy source with an abundant fuel supply. A promising approach to harnessing fusion power utilizes magnetic fields to confine a plasma with sufficient density and energy confinement time to achieve sustained thermonuclear temperatures, exceeding 100 million degrees Celsius for a fusion reactor fuelled by the hydrogen isotopes: deuterium (D) and tritium (T) [1] , [2] . The most advanced approach for magnetic confinement fusion is a doughnut-shaped confinement system known as a Tokamak [3] , as evidenced by a joint international effort in building a major next-step facility, international thermonuclear experimental reactor (ITER; http://www.iter.org ), to demonstrate scientific viability and some essential technologies for a fusion reactor. Anticipating scientific and technological successes of ITER, economic viability, ease of maintenance and safety should advance to the forefront of fusion energy development towards ultimate commercial use. The field-reversed configuration (FRC) is a simple compact toroid (CT) magnetic confinement system, that is, one without toroidal coils linking the plasma [4] , [5] , and thus with predominantly poloidal fields. The attractions of such a configuration for a potential fusion reactor are its simple, linear geometry for ease of construction and maintenance, as well as a natural, unrestricted divertor configuration for facilitating energy extraction and fusion ash removal. The FRC is a diamagnetic entity with current flowing across the magnetic field lines. Having no appreciable toroidal magnetic field greatly reduces the threat of dangerous disruptive events associated with massive magnetic energy and runaway electrons [6] , a great challenge facing fusion reactors. In addition, of all magnetic confinement systems, the FRC exhibits the highest β , defined as the ratio of the plasma pressure to the magnetic energy density of the externally supplied magnetic fields, approaching 100%, thus allowing for efficient use of magnet hardware. The high- β property also allows the use of advanced fusion fuels [7] , [8] . These features, coupled with its unique linear exhaust capability, also make the FRC a highly attractive candidate vehicle for deep-space explorations [9] . In the following, we report on a kinetic effect to stabilize a highly disruptive instability for an FRC, known as a tilt mode, provided by fast ions from energetic beam injection. The tilt mode is manifested as a spontaneous relaxation event marked by the abrupt ejection of a fraction of plasma from the confined region. The instability can be prevented altogether at a sufficient fast particle concentration. Another new finding is that active wall conditioning with titanium or lithium gettering to control edge neutrals and impurities is imperative for maintaining FRC stability by preventing density rise during the discharge. Such a stabilizing effect from fast particles, combined with the synergistic effect of the active boundary control, enables achievement of a fully-stable FRC scenario with a long lifetime. C-2 CT-merging FRC experiment Spectacular progress has been made on both physics and technology fronts of FRC development in the C-2 CT-merging FRC experiment ( Fig. 1 ) [10] , [11] , [12] , [13] , an effort entirely funded by private resources. It has recently achieved a long-lived FRC regime, with a marked improvement in confinement over one order of magnitude, departing from the predictions based on the scaling law in the previous experiments [14] . 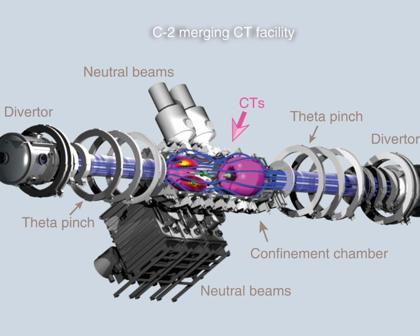Figure 1: Schematic of C-2 merging CT facility. C-2 system consists of a centre stainless-steel confinement vessel, two theta-pinch formation sections on opposite sides of the confinement chamber, and two divertors at both ends, with total axial span of∼20 m. There are eight neutral beams, three on each side of the confinement chamber and two on top of the confinement chamber for current drive and heating. Two plasma guns are located near the axial ends of the machine for active control of edge plasma. Figure 1: Schematic of C-2 merging CT facility. C-2 system consists of a centre stainless-steel confinement vessel, two theta-pinch formation sections on opposite sides of the confinement chamber, and two divertors at both ends, with total axial span of ∼ 20 m. There are eight neutral beams, three on each side of the confinement chamber and two on top of the confinement chamber for current drive and heating. Two plasma guns are located near the axial ends of the machine for active control of edge plasma. Full size image C-2 has adopted a collision-merging FRC formation scheme [15] , [16] , [17] by colliding two high- β CTs at a supersonic speed, each formed by a conventional theta-pinch [10] , [11] , producing high-temperature FRCs with radius r s ∼ 0.35 m, length , density n e ∼ 5 × 10 19 m −3 , total temperature T t = T i + T e up to 1 keV, external magnetic field, B e ∼ 0.1 T, plasma current I p ∼ 0.5 MA, , as expected for an FRC. The merged FRCs are centred in a metallic cylindrical confinement chamber of radius 0.7 m and length 5 m with strong magnetic mirrors (mirror ratio ∼ 3) at the cone-shaped ends of the chamber. The ultimate goal of C-2 is to achieve fusion-relevant FRC plasmas and explore their sustainment by neutral beam injection (NBI). The 20 keV hydrogen beams are injected tangentially into the confinement chamber with an impact parameter of 0.2 m before the FRC merging process. In view of the low internal magnetic field, the orbits of fast ions generated by NBI extend well outside the magnetic separatrix. This makes it essential to limit the edge neutral density to minimize fast-ion losses via charge exchange with cold neutrals [18] . Towards this end, an extensive effort of wall conditioning, using titanium gettering and advanced lithium-coating techniques, reduced both the neutral concentration in the edge plasma (well below 0.1%) and impurity radiation. In addition, we have demonstrated an active means of improving the stability and confinement property of the merged FRC as a suitable target plasma for NBI by applying line-tying and boundary-plasma biasing with plasma guns at the end divertors [12] , [13] . The former provides a restoring force that facilitates the centring of the plasma and reduces the off-centre ‘wobble’, while the latter produces an inward electric field E r with the E r × B z drift opposing the ion diamagnetic drift B z × ∇ p , thus reducing bulk plasma rotation. This proves effective at suppressing the magneto-hydrodynamic (MHD) instability with azimuthal mode number l =2 (the disturbance has the factor e ilθ where θ is the azimuth angle), which is driven by centrifugal forces developed from plasma rotation [4] , [5] . The end-electric biasing is also effective at suppressing edge fluctuations, thus improving confinement. Achievement of long-lived FRCs Coupling these active boundary control techniques with NBI, we have achieved long-lived FRCs, with the lifetime approaching 5 ms, far beyond the conventional theta-pinch-formed FRCs [4] , [14] , [19] , [20] , as shown in Fig. 2 . Here, the lifetime is defined as the time interval before the plasma radius falls to zero. Without NBI FRCs quickly disrupt with a much shorter lifetime and exhibit large shot-to-shot variations. Actually, the particular time trace shown in the figure for the case without NBI is averaged over a large number of discharges under the same operating conditions. This achievement clearly demonstrates NBI as an essential component for attaining FRC stability, against the potential l =1 tilt mode [21] , which has cast a great shadow over FRC development to date [4] , [5] . In common stability parlance the tilt is the lowest-order kink mode, but, unlike rotational modes, it is largely an internal disturbance in elongated FRCs with primarily an axial shift. The tilt is predicted to be the most dangerous instability of all by MHD theory because its ideal growth time is extremely short with 1/ γ mhd ∼ 5 μs for typical C-2 FRCs, which can lead to the destruction of FRC topology. Here, is the predicted growth rate of the ideal tilt instability with being the FRC length, being the Alfven speed based on the external magnetic field and the average density ( m i is the ion mass and μ 0 is the free-space permeability). Despite this fast ‘self-destruct’ rate, past FRCs usually survived a few dozen times longer than 1/ γ mhd (ref. 5 ), commonly ascribed to the highly kinetic nature of FRCs [22] , [23] , [24] , [25] , [26] and two-fluid effects [27] , [28] , [29] ; other stabilizing influences may have contributed in past experiments as well: sheared flow [30] ; small toroidal fields [20] , [31] , [32] , [33] ; and rotating magnetic fields [34] , [35] . 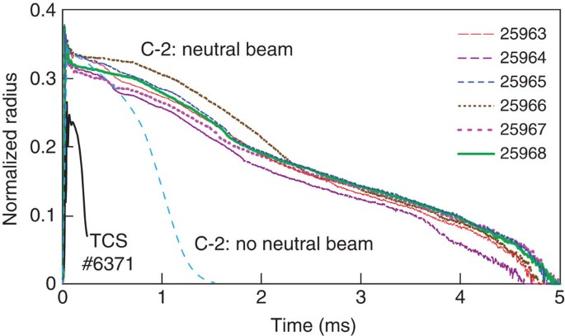Figure 2: Demonstration of long-lived FRCs with a lifetime far beyond conventional theta-pinch formed FRCs by neutral beam injection. Shown here are the time histories of the normalized excluded flux radius, which approximates the confined plasma radius,rΔφ∼rs, for a series of consecutive discharges obtained in C-2 with neutral beams, along with that averaged over a number of similar discharges without neutral beams. Also shown is a typical FRC obtained from the translation, confinement and sustainment (TCS) FRC experiment19,20, one of the previous longest-lived FRCs. (Errors for the magnetic measurements are <5%.). Figure 2: Demonstration of long-lived FRCs with a lifetime far beyond conventional theta-pinch formed FRCs by neutral beam injection. Shown here are the time histories of the normalized excluded flux radius, which approximates the confined plasma radius, r Δ φ ∼ r s , for a series of consecutive discharges obtained in C-2 with neutral beams, along with that averaged over a number of similar discharges without neutral beams. Also shown is a typical FRC obtained from the translation, confinement and sustainment (TCS) FRC experiment [19] , [20] , one of the previous longest-lived FRCs. (Errors for the magnetic measurements are <5%.). Full size image Stabilizing effects from neutral beam injection The highly kinetic property causes the ion and magnetic disturbances to get out of phase, which can stabilize or at least greatly reduce the growth rate [22] , [36] . NBI creates a large-orbit ion population, which potentially contributes to the kinetic effects, thus providing additional stability, but it has never been demonstrated before. We have employed the hybrid kinetic MHD (HKMHD) model in the 3D NIMROD code [37] to examine possible stabilizing effects of NBI to the l =1 tilt mode. In these simulations, the fast ion component (arising from NBI) is represented as a collisionless species using a particle-in-cell technique, with the bulk plasma being treated as an MHD fluid. The fast particle motion is coupled to the background fluid only through its influence on the magnetic field [24] . Thus, the thermal fluid equation of motion and resistive Ohm’s law remain the same but the Ampere’s law is adjusted as , where J is the thermal fluid current (ions+electrons), J b is the current driven by the fast particles from neutral beams, B is the magnetic field and μ 0 is the permeability of free space. For simulations with C-2 like parameters, the code predicts that without NBI the l =1 tilt mode grows and quickly disrupts the configuration within a few Alfvén times, as shown in Fig. 3 . In contrast, the growth of the simulated tilt mode can be suppressed at a ratio of the fast-particle to thermal-ion density n b / n i ∼ 7%, which is largely consistent with the experimental observations. For typical equilibrium FRCs after the merging formation process in C-2, the plasma contains ∼ 10 19 ions and ∼ 10 18 fast particles from NBI, hence, the fast particle concentration n b / n i ∼ 10%. Note, however, that the fast particle pressure is of similar order of magnitude to the thermal plasma pressure. This implies that high-energy beams will be needed for a reactor because of much higher plasma pressure. This awaits further investigation by taking into account contribution from fusion products such as alpha particles. 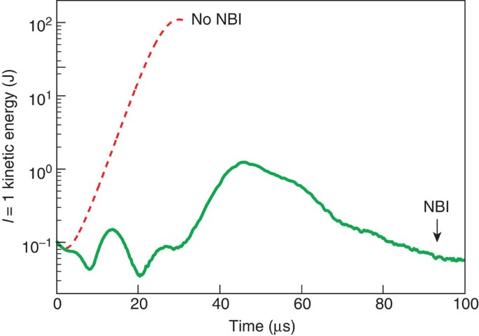Figure 3: Stabilizing effects from fast ions arising from NBI. The growth of the kinetic energy of the tilt mode predicted by the HKMHD/NIMROD code for a typical C-2 equilibrium with a fast particle concentrationnb/ni=7% (NBI), in comparison with the case withnb/ni=0 (no NBI). Figure 3: Stabilizing effects from fast ions arising from NBI. The growth of the kinetic energy of the tilt mode predicted by the HKMHD/NIMROD code for a typical C-2 equilibrium with a fast particle concentration n b / n i =7% (NBI), in comparison with the case with n b / n i =0 (no NBI). Full size image HKMHD/NIMROD modelling shows that the tilt mode leads to an axial shift with a significant ( l =1) perturbation to the radial magnetic field B r at the FRC ends, while the beam current maintains a dominant azimuthal component to J b in this region owing to large-orbit kinetic effects. This leads to an effective axial < J b, θ × B r > restoring force, hence providing a stabilizing effect on the tilt mode, as originally demonstrated numerically by Barnes and Milroy [24] . It is worth noting that, for the calculations shown in Fig. 3 , the l =1 mode is unstable for the initial beam parameters, but as the mode starts to grow it causes the beam to spread axially. That is the beam adjusts itself due to the perturbation, and after this adjustment the beam is more stabilizing, and the mode then decays. Another important finding for the achievement of the stable long-lived FRC scenario is the need for advanced wall conditioning with titanium gettering or lithium coating. In addition to improving NBI coupling to the FRC, as aforementioned, this also reduces recycling and impurity production resulting from plasma–wall interactions to avoid an unwanted growth in the density and consequent rise in S* for maintaining stability. where is the ion skin depth (a measure of the ion orbit size at high- β ); it measures the degree to which the plasma reacts like a fluid (high S* ) or an orbit-dominated (low S* ) object. An uncontrolled rise in plasma density tends to cause onset of a spontaneous transition midway through the discharge, which appears to be driven by the tilt mode (as discussed later), degrading the performance, even prematurely terminating the configuration. As shown in Fig. 4 , the transition event is manifested as an abrupt drop in the excluded flux radius r Δ φ . The excluded flux radius is r Δ φ ≡(Δ φ / πB e ) 1/2 , where Δ φ is the excluded magnetic flux as measured by a probe array arranged along the length of the confinement chamber. The r Δ φ in the figure is the maximum value, which is always near the axial midplane ( z =0). It represents the radius of the confined plasma on the closed magnetic field lines, approximating the magnetic separatrix radius, r Δ φ ∼ r s . The change in r Δ φ has a major implication, as the poloidal flux φ p is strongly dependent on r Δ φ . Recall that φ p is generated entirely by the cross-field plasma current. In contrast to other magnetic confinement systems, in FRCs the poloidal flux typically decays on the resistive timescale, closely inter-coupled to the cross-field transport rate. Thus, the abrupt (<0.1 ms) drop of r Δ φ during the transition marks a magnetic-reconnection event that annihilates a fraction of the poloidal flux. Simultaneous with it is a crash in the average density ( Fig. 4b ) and a rapid increase in the apparent plasma length ( Fig. 4e ). An integral part of this major restructuring is the ejection of a fraction of the plasma, as witnessed by the radiation bursts at the FRC ends immediately following the transition ( Fig. 4c , d ), detected by the bolometers located at z =±1 m from the midplane. The time delay is about 80 μs between the onset of the transition, as manifested by a spontaneous decrease in r Δφ , and the bursts of radiations at the FRC ends, commensurate with a jet velocity of ∼ 12 km s −1 . This is reminiscent of the ejecta from astrophysical jets and coronal mass ejections [38] , [39] , [40] , [41] . Incidentally, relaxation has also been observed during dynamic FRC formation processes [10] , [11] , [19] , suggesting the tendency towards a preferred plasma state in these high- β systems, just as is well known in some low- β laboratory plasmas [42] , [43] , [44] , [45] , [46] , [47] . 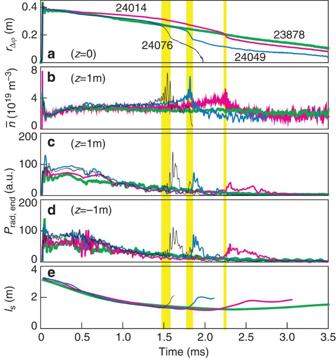Figure 4: Spontaneous transition during long-lived FRCs with NBI. The time traces of a series of discharges with and without transition. Data shown are the excluded flux radius,rΔφ, the line averaged electron density,, at the midplane of FRC,z=0, the radiated power atz=±1 m from the midplane,Prad,end, and the length of FRC,. Yellow shading indicates the time when the transition occurs for shots 24014, 24049 and 24076. (The lowest limit for the line-integrated density measurement is 0.3 × 1019m−2, and the absolute responsivity of bolometers varies between −30 and +50%, dependent on the photon energy.) Figure 4: Spontaneous transition during long-lived FRCs with NBI. The time traces of a series of discharges with and without transition. Data shown are the excluded flux radius, r Δ φ , the line averaged electron density, , at the midplane of FRC, z =0, the radiated power at z =±1 m from the midplane, P rad,end , and the length of FRC, . Yellow shading indicates the time when the transition occurs for shots 24014, 24049 and 24076. (The lowest limit for the line-integrated density measurement is 0.3 × 10 19 m −2 , and the absolute responsivity of bolometers varies between −30 and +50%, dependent on the photon energy.) Full size image Of particular importance is that the internal tilt mode usually leads to reconnection and annihilation of internal magnetic fields and hence termination of FRC. With application of neutral beam injection, the plasma usually relaxes into another FRC equilibrium, albeit with a lower internal magnetic flux, for typical FRC conditions in C-2. Moreover, this can be completely avoided while leveraging the synergistic effect from active boundary control, as demonstrated in Fig. 4 . The key parameters affecting tilt instability are S* and the elongation of the separatrix (ref. 5 ). 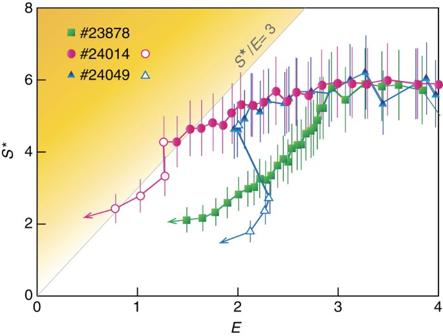Figure 5: Progression of FRC towards tilt instability boundaryS*/E∼3. The results are obtained from the three beam-driven long-pulse discharges shown in the previous figure. The solid and open symbols represent the data points before and after transition, respectively, with the arrows indicating time evolution of the discharges. The error bars represent the s.d. of the measurements. Figure 5 shows the trajectory of S* / E in the long-pulse discharges shown in the previous figure discussed above, where r s is approximated by r Δ φ and is estimated from excluded-flux-array measurements. We can see that, for the cases with transition, as the FRC elongation, E , dwindles (shots 24014, 24049), the FRC proceeds towards a higher S */ E value, finally approaching the instability boundary with S */ E ∼ 3, as expected from the tilt theory. It is worth noting that as the elongation increases on relaxation, the plasma rebounds from the instability boundary, as predicted by tilt stability theory and verified by extensive modelling [5] . It then restructures into a new state, staying safely away from the transition. No other instabilities that have been identified for FRCs until now can explain these observations. Figure 5: Progression of FRC towards tilt instability boundary S */ E ∼ 3. The results are obtained from the three beam-driven long-pulse discharges shown in the previous figure. The solid and open symbols represent the data points before and after transition, respectively, with the arrows indicating time evolution of the discharges. The error bars represent the s.d. of the measurements. Full size image The physics process of the relaxation driven by tilt is illustrated by HKMHD/NIMROD modelling, as shown in Fig. 6 . As the FRC elongation E shrinks, the pressure profile peaks near the midplane ( Fig. 6a ), and the FRC becomes unstable to the tilt mode. The tilt mode leads to a significant perturbation in the plasma pressure profile, much larger than the magnetic perturbation. Clearly, the pressure profile exhibits an axial displacement, as manifested by the shifts in the bright spots in Fig. 6b . The code predicts that the beam current perturbation is out of phase with the plasma pressure perturbation. This, in turn, reduces the growth of the tilt mode, and the plasma enters a new stable and quiescent equilibrium state. In particular, the modelling shows that the pressure profile expands axially during the relaxation, leading to an increase in the elongation, E , to steer away from the instability cliff to reach the final relaxed state ( Fig. 6c ), in agreement with the experiments. 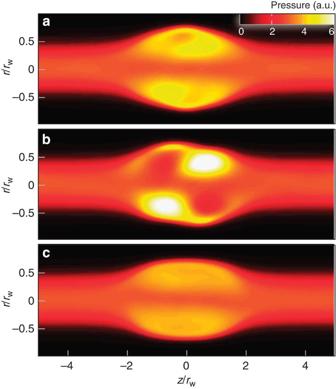Figure 6: 3D HKMHD/NIMROD reproduces the FRC transition. Contours of plasma pressure in an FRC with a relatively small fast particle concentration from NBI, obtained from HKMHD/NIMROD calculations. (a) In the equilibrium phase before the development of the tilt mode. (b) During the tilt mode at maximum perturbation. (c) In the new quiescent state after tilt perturbation decays away. Figure 6: 3D HKMHD/NIMROD reproduces the FRC transition. Contours of plasma pressure in an FRC with a relatively small fast particle concentration from NBI, obtained from HKMHD/NIMROD calculations. ( a ) In the equilibrium phase before the development of the tilt mode. ( b ) During the tilt mode at maximum perturbation. ( c ) In the new quiescent state after tilt perturbation decays away. Full size image A central obstacle to FRC development is its stability to the MHD instabilities with low azimuthal mode numbers, that is, l =1 tilt mode and l =2 rotational mode [4] . The stability of the l =2 rotational mode has been achieved by applying various control techniques, for example, external static fields [4] , rotating magnetic fields [34] and the plasma gun [12] , [13] . However, active stabilization of the most dangerous l =1 tilt mode has not been demonstrated before this work. The tilt mode leads to tearing and annihilation/reconnection of the internal magnetic flux surface, and thus the loss of FRC magnetic configuration. We have demonstrated the stabilizing effect of fast ions by NBI, achieving a stable, high- β plasma state with a lifetime of about 5 ms. This achievement was enabled by the injection of energetic particles from NBI in concert with active plasma boundary control. These advances enhance the prospect of an economic fusion reactor with an extremely high β and simple geometry, thus providing a compelling additional platform for the development of economic fusion energy. The C-2 device The C-2 is an FRC facility that was designed to demonstrate FRC sustainment with the neutral beam injection for heating and current drive. The C-2 device consists of a central confinement vessel, interposed between two CT formation sections, and two divertor chambers at each end to control neutrals and impurities. Typical C-2 equilibrium FRC parameters are as follows: separatrix radius r s ∼ 0.4 m, separatrix length , external magnetic field B e ∼ 0.1 T, average density n e ∼ 5 × 10 19 m −3 , total temperature T t = T i + T e up to 1 keV and plasma current I p ∼ 0.5 MA. The C-2 is equipped with eight neutral beams distributed around the azimuth and along the central confinement vessel of the machine, and two plasma-guns mounted coaxially in each divertor. NB injection On the C-2 device NB injection offers a most principal means for FRC plasma heating, current drive and stabilization. Six NBs (20 keV, Hydrogen, 0.7 MW per unit) with total 4 MW power are routinely injected perpendicular to the confinement chamber and aimed tangentially in the FRC current direction (co-injection), with an impact parameter of 0.2 m. The C-2 FRC parameters are suitable for NB capture (Monte-Carlo simulations indicate that shine-through and first orbit losses less than 10%) and for fast ion confinement (slowing down time ∼ FRC lifetime). The fast ions, created by charge exchange, trace out large-scale betatron orbits that contribute to the plasma current and build up a fast-ion population with pressure eventually comparable to the thermal pressure. Plasma gun The plasma guns on C-2 are used to produce and direct plasma flows at high-energy densities. These plasma guns generate a warm (electrons T e ∼ 30–50 eV, ions T i ∼ 100 eV), tenuous ( n e <10 19 m −3 ) and annular (0.11 m inner diameter and 0.13 m outer diameter) plasma stream for about 6 ms. The typical anode-to-cathode voltage difference is ∼ 500 V, and the gun arc-current is ∼ 10 kA. The gun magnet provides an axial magnetic field ∼ 0.5 T. The plasma guns perform multiple functions (1) to create an inward radial electric field in the scrape off layer (SOL) (important for stabilizing n =2 rotational mode), (2) to establish electromagnetic shear in the SOL (effective to suppress local fluctuations) and (3) to tightly centre the plasma (less n =1 wobble motion) via line-tying to the gun electrodes. How to cite this article: Guo, H. Y. et al . Achieving a long-lived high-beta plasma state by energetic beam injection. Nat. Commun. 6:6897 doi: 10.1038/ncomms7897 (2015).